Biotechnological development of plants for space agriculture 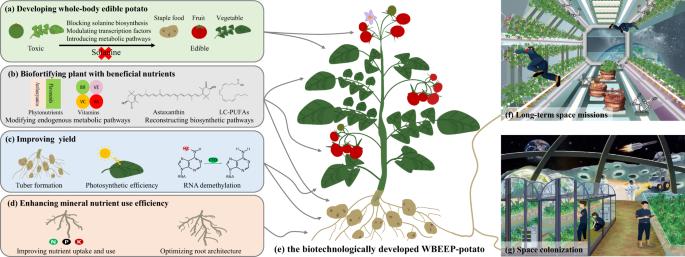Fig. 1: Biotechnological generation of WBEEP-potato and its applications. aDeveloping whole-plant edible potatoes. Blocking the biosynthesis of solanine, varying its transcriptional regulation, or introducing other metabolic pathways can reduce the accumulation of solanine and make potato stems, leaves and berries edible.bBiofortifying plants with beneficial nutrients. Biofortification can provide phytonutrients (e.g., flavonoids, anthocyanins, and carotenoids) by modifying endogenous metabolic pathways and astaxanthin or VLC-PUFAs (e.g., arachidonic acid) by reconstructing biosynthetic pathways.cImproving yield. Potato yield can be increased by improving tuberization, photosynthetic efficiency and RNA demethylation.dEnhancing mineral nutrient use efficiency. Nutrient utilization efficiency can be improved by modulating plant nutrient absorption, allocation and metabolism or optimizing root architecture.e–gThe biotechnologically developed WBEEP-potato (e) is expected to be applied in long-term space missions (f) and space colonization (g). Plants whose whole bodies are edible would be desirable for space farms because they can bring humans more food and reduce waste. However, potato stems, leaves, and berries are inedible. The aerial parts of potato plants contain accumulated solanine (primarily α-solanine and α-chaconine), which defends against pests and pathogens but is toxic to humans. In space farming systems, with highly controlled environments, solanine-mediated plant resistance would be unnecessary. If solanine were removed, the whole potato plant could potentially become edible. To block the accumulation of solanine in potato plants, biosynthesis can be targeted. For example, silencing or mutating genes encoding the cytochrome P450 enzyme GAME4, the dioxygenase DPS or the AP2/ERF transcription factor GAME9 greatly reduced solanine content [3] , [4] , [5] . Tomatoes can also produce toxic solanine (primarily α-tomatine) but can convert solanine into the nonbitter and nontoxic glycoside esculeoside A in fruits [6] . Since solanine metabolism involves several enzymatic reactions in common between potatoes and tomatoes, it might be possible to introduce solanine metabolism genes from tomatoes into potatoes to reduce solanine accumulation. Phytonutrients (e.g., flavonoids and anthocyanins) and vitamins are of great importance to human health. The body in space becomes more fragile and needs more nutrients [7] . However, several micronutrients in packaged foods are likely to break down under storage conditions in space, which makes it difficult for crews to obtain stable nutrients [8] . Therefore, it is desirable for people to obtain nutrition directly from fresh agricultural products. Considering the insufficient content of proteins, phytonutrients, vitamins, and other essential nutrients in potato tubers, it would be necessary to biofortify potatoes to fully meet the nutrient needs of the human body. Plants can be improved to synthesize vitamins and functional secondary metabolites by modifying endogenous metabolic pathways, including (1) increasing the precursor supply; (2) overexpression, relocation, or mutation of bottleneck enzymes; (3) silencing the undesired pathways; (4) blocking the competing pathways; (5) expansion of metabolic flow to reduce feedback inhibition; and (6) regulation of transcription factors. Through the application of the above strategies, potatoes that are rich in various vitamins, proteins, flavonoids, anthocyanins, and other nutrients have been developed [9] . Moreover, potato varieties containing canthaxanthin, astaxanthin, or very-long-chain polyunsaturated fatty acids (VLC-PUFAs) may be developed by reconstructing biosynthetic pathways [10] . Tubers are the primary edible parts of potato plants. Potato tuberization is a complex biological process. Key regulators include photoreceptor phytochrome B (PHYB), transcription factor StCO, mobile signals ( StBEL5 and POTH1 mRNA, StSP6A protein, and miR172 ), and sucrose transporters StSUT4 and StSP5G. Overexpression of StSP6A , StPOTH1 , StBEL5 , and StmiR172 or inhibition of StPHYB , StCO , StSUT4 , and StSP5G can be performed to improve tuberization [11] . Optimization of photosynthesis is one of the primary ways to increase crop yield, and potato tuberization also requires large amounts of photosynthetic products (especially sucrose) from the aboveground parts. Efforts are ongoing to increase photosynthetic efficiency by improving the carboxylation capacity of the Rubisco enzyme, enhancing the regenerative capacity of the carbon reduction cycle, optimizing the electron transport chain, and minimizing oxygenation and photorespiration [12] . Most of the abovementioned genetic engineering strategies for improving photosynthesis efficiency have been successfully applied in rice or tobacco and could hopefully be utilized to improve potato yield. For example, an artificially constructed photorespiratory bypass through the expression of a recombinant glycolate dehydrogenase polyprotein can significantly increase the photosynthetic efficiency and tuber yield by reducing photorespiration and improving CO 2 uptake [13] . Recently, modulating plant RNA m 6 A methylation has become an efficient way to improve plant growth and crop yield. Transgenic expression of the human RNA demethylase FTO to reduce m 6 A levels in potatoes led to ~50% increases in tuber yield and aerial biomass [14] . Crop growth and development require many mineral elements, including nitrogen, phosphorus, and potassium. The cost of transporting fertilizers from Earth is very high. Therefore, it is necessary to improve crop nutrient utilization efficiency to reduce fertilizer consumption. Genetic modification could be carried out to enhance plant nutrient absorption, allocation, and metabolism or to optimize root architecture [12] . Nitrogen is one of the most important elements required by plants. Glutamate dehydrogenases (GDHs) from lower organisms show a higher affinity for NH 4 + and a stronger ammonia assimilation ability. Heterologous expression of GDHs that have higher affinity for NH 4 + than plant GDHs can improve the nitrogen use efficiency of many crops, including potatoes, and ensure that crops can obtain high yields under low-nitrogen conditions [15] . Phosphorus is another essential element for plant growth, and phosphite fertilizers can promote an increase in the yield and quality of potato tubers. Expression of phosphite dehydrogenase ( ptxD ) from Pseudomonas spp. allows rice and cotton to metabolize phosphite in addition to phosphate [16] , and its role in potato is worth exploring. Potatoes need more potassium fertilizer than nitrogen or phosphate fertilizers for growth and quality. Heterologous expression of the Arabidopsis K + channel AKT1 and its activators CBL1 , CBL9 , and CIPK23 can increase the efficiency of potassium uptake from the soil in several crops, and overexpressing the K + transporter HAK5 may increase the efficiency of potassium uptake in many crops under potassium-limited conditions [17] . Recently, genetically manipulating the root system architecture has become an emerging strategy to increase nutrient acquisition and yield in tuber crops, but genes that can be exploited in potatoes must be mined. Experiments have been conducted to show how plants grow and develop in space, but clear space agriculture remains in its infancy. Only green leafy vegetables such as lettuce and mustard are currently grown for food on the International Space Station [18] . Thus, to bring more plants to space farms, we propose the WBEEP approach for crop improvement. A comprehensively applied WBEEP could provide sufficient and nutritious food for humans in space with minimal fertilizer consumption. As more anti-nutritional factor biosynthesis mechanisms are revealed, and strategies for improving nutrition, yield, and fertilizer use efficiency are developed, the WBEEP approach could be implemented on more crops. While the practical cultivation of WBEEPs in space for food might not be achievable any time soon, we suggest that considering the incremental advances needed to achieve such a goal might be beneficial not only for space agriculture but also for conventional agriculture.